Two centuries of limited variability in subtropical North Atlantic thermocline ventilation Ventilation and mixing of oceanic gyres is important to ocean-atmosphere heat and gas transfer, and to mid-latitude nutrient supply. The rates of mode water formation are believed to impact climate and carbon exchange between the surface and mid-depth water over decadal periods. Here, a record of 14 C/ 12 C (1780–1940), which is a proxy for vertical ocean mixing, from an annually banded coral from Bermuda, shows limited inter-annual variability and a substantial Suess Effect (the decrease in 14 C/ 12 C since 1900). The Sargasso Sea mixing rates between the surface and thermocline varied minimally over the past two centuries, despite changes to mean-hemispheric climate, including the Little Ice Age and variability in the North Atlantic Oscillation. This result indicates that regional formation rates of sub-tropical mode water are stable over decades, and that anthropogenic carbon absorbed by the ocean does not return to the surface at a variable rate. In the North Atlantic, ocean thermocline waters along the Gulf Stream (GS) are reintroduced into the surface layer, and waters within and south of the GS are subducted into the thermocline in what is commonly referred to as Sub-Tropical Mode Water or 18° Water (EDW) formation. This process leads to vigorous mixing of waters above and within the thermocline in large volumes [1] and is known to occur between 33°–40°N and 30°–75°W (ref. 2 ). By redistributing nutrients in the upper layers, EDW formation is believed to have a role in regulating the biogeochemical processes of the nutrient-limited subtropical gyre [3] , [4] by supplying nutrients to the surface. In addition, EDW formation contributes as much as 3–10% of the global net annual draw-down of anthropogenic CO 2 on intermediate time scales (10s–100s of years) [5] ; thus, changes to the rates of formation could alter the oceanic carbon sink. However, our understanding of the long-term variability of these ocean dynamics is still limited [6] . In the North Atlantic, EDW formation occurs as a result of vigorous surface ocean convection caused by rapid heat release from the ocean to the atmosphere, and perhaps also by local frontal instabilities within the GS [6] . The rate of mode water formation appears closely related to the phase of the North Atlantic Oscillation (NAO) [2] , [7] , [8] , [9] , the dominant mode of atmospheric variability in the region that is generally defined as the winter (December–March) atmospheric pressure difference between Iceland and the Azores [10] . In a negative phase of the NAO, the pressure difference weakens, slowing the speed of the atmospheric jet stream across the North Atlantic and increasing storminess off eastern North America. The increased storminess increases the air–sea heat exchange, thus increasing the rate of formation of EDW. As new EDW is formed during the winter, the colder, denser waters at the surface mix down into the thermocline that includes 'older' (lower 14 C) mode waters that have re-circulated around the subtropical gyre. When surface waters warm in spring, the mixed layer shoals and the water column re-stratifies, but some of the deeper 'older' thermocline water remains in the surface, effectively increasing the surface radiocarbon age. Thus, Δ 14 C (the per mil deviation of 14 C/ 12 C from that in nineteenth century wood) in the surface ocean can be used as a measure of ventilation (vertical mixing), because it represents the combination of dissolved inorganic carbon exchanging with atmospheric CO 2 and surface water mixing with deeper layers that have been isolated from atmospheric CO 2 . Previously in this region, past changes in ventilation were reconstructed back to 1880 from biennial, high-precision Δ 14 C measurements of a Bermuda coral taken near North Rock along the northern reef [11] ( Fig. 1 ). The study revealed significant variability in Δ 14 C (−50 to −35‰; Fig. 2 ) correlated to the NAO, with lower surface Δ 14 C occurring during periods of negative NAO phase associated with enhanced EDW ventilation. The record also demonstrated no 14 C Suess Effect, and a significant 13 C Suess Effect ( Fig. 2 ), which is the decrease in δ 13 C in the environment beginning in the late 1800s, and originating mostly from the combustion of fossil fuel and biomass whose δ 13 C values are much lower than that in the atmosphere. These combined results indicate that waters surrounding Bermuda are influenced by both vertical ocean mixing and atmospheric exchange. In this study, we aimed to extend the record into the end of the Little Ice Age to evaluate changes in mixing rates at times of cooler mean hemispheric temperature and lower NAO variability. We report biennial, high precision Δ 14 C time-series measurements from an annually banded coral from 1780 to 1940, collected from the Sargasso Sea along the south shore of Bermuda (64°W, 32°N; Fig. 1 ). The Δ 14 C time history of atmospheric CO 2 is well documented [12] as is the Δ 14 C time history of GS water [11] that supplies surface water to the Sargasso Sea, allowing us to evaluate past changes in ventilation. 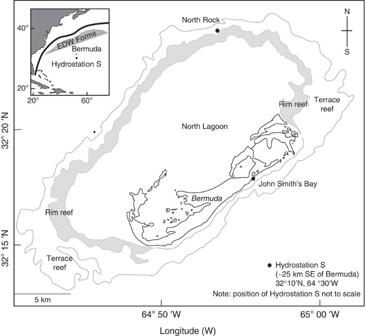Figure 1: Map of Bermuda within the North Atlantic subtropical gyre. Approximate locations of sampling sites North Rock and John Smith's Bay are indicated. The island of Bermuda is characterised by a large lagoon surrounded by a barrier reef to the north and a narrow shelf with barrier reef to the south. Inset shows Bermuda relative to an approximate region of 18° mode water (EDW) formation and the eastern coast of the United States. Map based upon figures in Palteret al.4and Bateset al.13 Figure 1: Map of Bermuda within the North Atlantic subtropical gyre. Approximate locations of sampling sites North Rock and John Smith's Bay are indicated. The island of Bermuda is characterised by a large lagoon surrounded by a barrier reef to the north and a narrow shelf with barrier reef to the south. Inset shows Bermuda relative to an approximate region of 18° mode water (EDW) formation and the eastern coast of the United States. Map based upon figures in Palter et al . [4] and Bates et al . 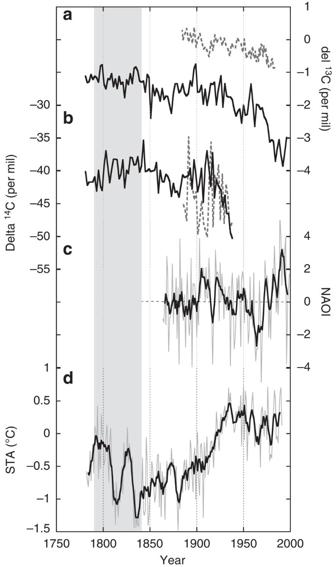Figure 2: Carbon isotope records from Bermuda and regional climate records. (a) Records of coral δ13C values from the north (dashed, Druffel11) and south (solid, this study) shore of Bermuda. (b) Coral Δ14C records for the north (dashed, Druffel11) and south (solid, this study) shore for the entire 200 years. Note increased variability in the north-shore coral. Measurement error of ±2.5‰ (1σ). (c) Instrumental record of the NAO annually (shaded) and 5-year running mean (solid) from Hurrel10including the 0-index line (dashed). (d) A multi-proxy record of Northern hemisphere surface temperature anomalies (STA) including mean annual (shaded) and 5-year running mean (solid) from Joneset al.16Shaded area represents the Dalton Minimum in solar activity. [13] Full size image Figure 2: Carbon isotope records from Bermuda and regional climate records. ( a ) Records of coral δ 13 C values from the north (dashed, Druffel [11] ) and south (solid, this study) shore of Bermuda. ( b ) Coral Δ 14 C records for the north (dashed, Druffel [11] ) and south (solid, this study) shore for the entire 200 years. Note increased variability in the north-shore coral. Measurement error of ±2.5‰ (1σ). ( c ) Instrumental record of the NAO annually (shaded) and 5-year running mean (solid) from Hurrel [10] including the 0-index line (dashed). ( d ) A multi-proxy record of Northern hemisphere surface temperature anomalies (STA) including mean annual (shaded) and 5-year running mean (solid) from Jones et al . [16] Shaded area represents the Dalton Minimum in solar activity. Full size image Carbon isotope records from Bermuda The coral data show similar decadal to centennial scale behaviour as the atmospheric record of Δ 14 C ( Fig. 3 ). Biennial Δ 14 C coral measurements from 1780 to 1925 have no apparent trend; though measurements from 1926 to 1940 have a substantial decreasing trend with a low value of −50‰ (range before 1926 is −44 to −35‰), which we attribute to the Suess Effect. In addition, the coral Δ 14 C record has a significant linear correlation to the record of atmospheric Δ 14 C with a 10-year lag [14] , matching the time scale over which the surface ocean and atmosphere CO 2 mix, ( r =0.62, P ≪ 0.0001, n =72). Cross-spectral analysis of the two records confirms that they are significantly correlated for frequencies lower than 0.12 cycles per year (8-year period and longer) at a 95% confidence interval ( Fig. 3b,c ). The agreement between the coral and atmosphere Δ 14 C records implies that surface waters south of Bermuda are influenced predominantly by atmospheric exchange. 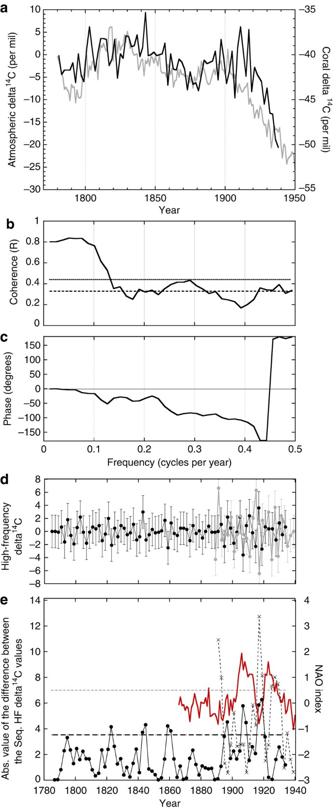Figure 3: Influences on and variability of oceanic Δ14C. (a) Record of atmospheric Δ14C (Stuiver and Quay12; shaded) and the south-shore coral Δ14C (solid). The correlation coefficient between the two records is 0.62 (P≪0.0001), with the coral record lagging the atmospheric record by 10 years. (b) Cross-correlation analysis of the south-shore coral and atmospheric Δ14C reconstructions (solid). Confidence levels (80%) are shown by the dashed line and 95% confidence level by dotted line. (c) Phase lag between the south-shore coral and atmospheric Δ14C reconstructions. (d) A 5-box Hanning filter was applied to the Δ14C records to isolate all frequencies higher than 10 years per cycle. The high-frequency record is plotted versus time for this study (solid) and Druffel11(shaded). Measurement error of ±2.5‰ is shown for each data point. (e) The absolute (Abs.) value of the difference between each sequential (Seq.) sample pair in the high-frequency (HF) record is plotted versus time for this study (solid dots) and Druffel11(shaded crosses). Propagated measurement error of ~3.5‰ (1σ) is shown by the solid dashed line and 2σ (~7.0‰) is shown by the shaded dashed line. Relatively few points show statistical independence (that is, above the measurement error) particularly for this study. The 5-year running mean of the instrumental record of the NAO index is shown in red10. Figure 3: Influences on and variability of oceanic Δ 14 C. ( a ) Record of atmospheric Δ 14 C (Stuiver and Quay [12] ; shaded) and the south-shore coral Δ 14 C (solid). The correlation coefficient between the two records is 0.62 ( P ≪ 0.0001), with the coral record lagging the atmospheric record by 10 years. ( b ) Cross-correlation analysis of the south-shore coral and atmospheric Δ 14 C reconstructions (solid). Confidence levels (80%) are shown by the dashed line and 95% confidence level by dotted line. ( c ) Phase lag between the south-shore coral and atmospheric Δ 14 C reconstructions. ( d ) A 5-box Hanning filter was applied to the Δ 14 C records to isolate all frequencies higher than 10 years per cycle. The high-frequency record is plotted versus time for this study (solid) and Druffel [11] (shaded). Measurement error of ±2.5‰ is shown for each data point. ( e ) The absolute (Abs.) value of the difference between each sequential (Seq.) sample pair in the high-frequency (HF) record is plotted versus time for this study (solid dots) and Druffel [11] (shaded crosses). Propagated measurement error of ~3.5‰ (1σ) is shown by the solid dashed line and 2σ (~7.0‰) is shown by the shaded dashed line. Relatively few points show statistical independence (that is, above the measurement error) particularly for this study. The 5-year running mean of the instrumental record of the NAO index is shown in red [10] . Full size image Similarly, the coral δ 13 C data from this study exhibit a 13 C Suess Effect with values decreasing 0.013‰ per year (±0.002) over 1885–1978 ( Fig. 2 ), in agreement with an average of coral records from around the globe [15] . The coral δ 13 C data show a gradual decline early in this period, with a much sharper decline from the 1960s onward, consistent with many corals in the Atlantic Basin [15] ( Fig. 2 ). Δ 14 C variability North and South of Bermuda This study from south Bermuda shows less Δ 14 C variability than the North Rock coral record previously reported [11] , with values from 1880 to 1910 ranging from −44 to −35‰ versus −50 to −35‰ for the southern and northern corals, respectively ( Fig. 2 ). The south-shore coral has approximately 50‰ less variability (results of F -test for variance, P =0.06, n =27) than the North Rock coral [11] , which shows abrupt negative excursions interpreted as times of increased ventilation and injection of older thermocline waters into the surface layer. The contrasting signals between the corals indicate that the two locations are experiencing different apparent rates of ocean mixing. Previous studies document that south-shore corals more accurately represent Hydrostation S, a 50-year hydrographic station located 25 km southeast of Bermuda ( Fig. 1 ), than do corals from North Rock [17] , [18] . Differences between the north and south have been found in sea surface temperature (SST) records generated from coral Sr/Ca that are attributed to differences in coastal circulation [19] . Studies from the north reef have found agreement between seasonal variations in coral Sr/Ca and SST data from Hydrostation S; however, there is no relationship between North Rock Sr/Ca and SST at interannual timescales (that is, comparing data for wintertime only) [19] , [20] . This indicates that the Sr/Ca to SST correlation is driven by the seasonal cycle that occurs each year in both records rather than the North Rock Sr/Ca accurately capturing inter-annual ocean conditions in the southern and central Sargasso Sea. In contrast, the Sr/Ca record from the south-shore coral used here shows strong relationships to Hydrostation S SST at both annual (seasonal cycle) and interannual (wintertime) timescales [17] , [18] ( Fig. 4 ). In addition, a strong correlation has been established between south-shore coral wintertime Sr/Ca and the NAO at varying frequencies [21] . These results indicate that the south-shore coral more accurately reflects conditions at Hydrostation S, and thus the open ocean conditions in the southern and central Sargasso Sea. The difference between the response of Δ 14 C to NAO variability at the two locations likely lies in enhanced local upwelling along the north reef because of the trade winds, which shift north to Bermuda during periods of negative NAO. Simultaneously, water formed due to enhanced EDW formation to the north of Bermuda will be advected southward, forming a large wedge of significantly 'older' water just below the seasonal thermocline around Bermuda. These subsurface waters are therefore upwelled along the north but not the south shore, reducing only north Bermuda Δ 14 C during negative NAO phases. This Δ 14 C signal will be limited to the waters north of Bermuda as a function of local topography, rather than occurring throughout the southern and central Sargasso Sea. 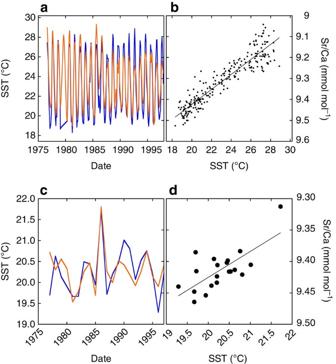Figure 4: South-shore coral Sr/Ca and Hydrostation S SST from 1976 to 1997. The data is shown at both monthly for the full seasonal cycle (top two panels) and winter average (December–March) (bottom two panels) timescales and is shown versus time and linearly. (a) Monthly Sr/Ca (orange) and Hydrostation S SST (blue) versus time, (b) monthly Sr/Ca and Hydrostation S SST linearly regressed (r2=0.86,P=0.0001). (c) wintertime Sr/Ca (orange) and Hydrostation S SST (blue) versus time, (d) winter average Sr/Ca and Hydrostation S SST linearly regressed (r2=0.51,P=0.0004). Figure adapted from Goodkinet al.17 Figure 4: South-shore coral Sr/Ca and Hydrostation S SST from 1976 to 1997. The data is shown at both monthly for the full seasonal cycle (top two panels) and winter average (December–March) (bottom two panels) timescales and is shown versus time and linearly. ( a ) Monthly Sr/Ca (orange) and Hydrostation S SST (blue) versus time, ( b ) monthly Sr/Ca and Hydrostation S SST linearly regressed ( r 2 =0.86, P =0.0001). ( c ) wintertime Sr/Ca (orange) and Hydrostation S SST (blue) versus time, ( d ) winter average Sr/Ca and Hydrostation S SST linearly regressed ( r 2 =0.51, P =0.0004). Figure adapted from Goodkin et al . [17] Full size image The agreement with atmospheric Δ 14 C and Hydrostation S, and the lack of negative excursions in Δ 14 C in the south-shore record brings into question whether there has been a detectable change to the mixing rate of surface and thermocline waters over the past 200 years. To investigate this, we employed a 5-box Hanning filter to remove all frequencies lower than 0.10 cycles per year (>10-year period), when the Δ 14 C is clearly driven by atmospheric exchange. With few exceptions, the difference between individual pairs of sequential biennial samples does not exceed the measurement error, indicating that high-frequency changes in Δ 14 C due to variable mixing rates, if present, are likely small and not well resolved from the coral data ( Fig. 3d,e ). That is, a measurable rate of change to vertical mixing is not present within the precision limits of the 14 C data. Between 1900 and 1920, there is a period when both this new coral record from the south shore and the earlier record from North Rock exhibit multiple sample pairs with significant changes to Δ 14 C above measurement error. These data correspond to a time of extended positive NAO with a short, but sharp, negative excursion around 1915, when changes to NAO-driven mode water formation rates would be high. However, cross-correlation analysis between the entire record of the raw Δ 14 C values presented here and the instrumental record of the NAO [10] shows no significant correlation at high or low frequencies. Low Δ 14 C variability along the south shore is also seen during the end of the Little Ice Age from 1800 to 1870, when SSTs are low [22] and NAO variability is weak [21] . In summary, surface waters to the south of the Bermuda exhibit a significant atmospheric 14 C imprint and minimal changes through time in the mixing rate with older subsurface waters, despite significant changes to NAO behaviour [21] and mean hemispheric climate [16] ( Fig. 2c,d ). Time scales for horizontal circulation in the Sargasso Sea, the tight recirculation component of the anticyclonic subtropical gyre, are believed to be on the order of 5 years [1] , [23] , indicating that surface waters are relatively well mixed over the sampling resolution of the coral records (2 years). Using transient tracers, Jenkins [24] determined that advection along isopycnals contributes significantly to thermocline ventilation within the Sargasso Sea. Studies evaluating water mass renewal rates in the Sargasso Sea yield tracer-based renewal time scales for the upper thermocline from a few years to a few decades, with slower renewal rates for the deeper isopycnal layers [11] , [23] , [25] , [26] . To calculate the water mass renewal rate within the Sargasso Sea, we employ a 5-box model based upon the model previously presented in Druffel [11] and similar to Druffel [25] . The five boxes are: the surface Sargasso Sea as represented by Bermuda ( B ), the atmosphere ( A ), slope water ( S ), GS water and subsurface water ( D ; Fig. 5 ). 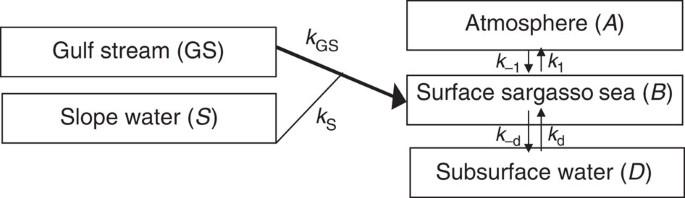Figure 5: Schematic showing the interactions of the 5-box model. Boxes include the atmosphere (A), Surface Sargasso Sea (B), Subsurface water (D), the Gulf Stream (GS) and Slope water (S). The rate of change of the surface reservoir for 14 C at B involves the balance of the air–sea gas exchange, and lateral and vertical seawater flux, which can be described as: Figure 5: Schematic showing the interactions of the 5-box model. Boxes include the atmosphere ( A ), Surface Sargasso Sea ( B ), Subsurface water ( D ), the Gulf Stream (GS) and Slope water ( S ). Full size image where d B /d t is the time rate of change in Sargasso Sea surface layer 14 C, lateral netflux is the combined net exchange with slope water ( S ) and the GS, and vertical netflux is the net exchange due to exchange with the thermocline ( D ). This can be written more explicitly as: where 0.983 is the isotopic fractionation factor when 14 CO 2 is transferred from the atmosphere to surface waters [27] , and A , B , GS, S and D are Δ 14 C values for the respective reservoirs based on 14 C/ 12 C ratio measured on environmental proxies. Measured coral Δ 14 C from Bermuda (this study) and from Florida [11] (Pickles Reef) are used for B and GS, respectively. The pre-bomb Δ 14 C for S is set to −71‰ [28] , [29] , [30] , [31] ( http://calib.qub.ac.uk/marine ). It is important to note that both the GS and S water are sources of low Δ 14 C to B before bomb testing, but GS during the peak years of the bomb era (1960s) is found to be higher than B [25] . The atmospheric box's (A) Δ 14 C values are set equal to tree-ring values [12] . The Δ 14 C for D is −50.6‰, a weighted average of pre-bomb 14 C data over the thermocline [32] . The exchange rates between each box and the surface box taken with respect to the volume of the surface box are k −1,GS,S,D ; k d is unknown; k GS and k S are set at 0.1275 and 0.0225 per year, respectively [26] . Atmospheric flux is described as: where CO 2 (aq) is dissolved CO 2 (0.019 mol m −3 ), ΣCO 2 is the total dissolved inorganic carbon (or total CO 2 ) in surface waters (2.12 mol m −3 ), Z is the annual-average mixed layer depth of the surface ocean (taken as 135 m in this region), and V p is a function of wind speed (WS) such that: from Jenkins [33] and Roether [34] with an average annual wind speed of 6.2 m s −1 . Assuming a pre-industrial steady state for equation (2) allows us to solve for k d : Average values for 1890–1910 14 C levels in the model reservoirs ( R / R 0 , ratio of sample 14 C/ 12 C to reference R 0 ) are B =0.9599 (−40.1‰), A =0.9959 (−4.1‰), GS =0.9512 (−48.8‰), S =0.9290 (−71.0‰) and D =0.9494 (−50.6‰). Therefore, we find k d to be 0.16 per year or 16% of the surface box volume per year. An error estimate for the exchange rate k d of ±0.10 (1 sigma) is found by error propagation using standard methods [35] . For B , A and GS, we use the s.e. calculated of measurements made between 1890 and 1910. As B and A are known to co-vary, the error was propagated using a combined error for (A/0.983-B). For S and D , we assume an s.e. to be the average of that for GS and B (0.8‰). The error estimate for k d is likely smaller than the true error, because it neglects error terms in the exchange rates. The volume of the Sargasso Sea surface layer is approximately 9.5×10 14 m 3 assuming a mixed layer depth [11] of 135 m. If the ventilation rate is 16% per year, then the annual amount of water exchanged would be 1.6×10 14 m 3 per year or approximately 5 Sv of continuous flow over a period of 1 year (Svy; 1 Sv=10 6 m 3 s −1 ; 1 Sv flow for 1 year (Svy) is equal to 3.154×10 13 m 3 ). These estimates are consistent with recent estimates of net annual EDW formation of 4.6 Svy [36] . The limited interannual variability in the south-shore coral Δ 14 C record can be used to place a bound on water mass renewal rate variability as well. With a measurement error of ±2.5‰ (1σ), the difference between two adjacent samples would need to exceed ±3.5‰ (1σ; assuming independent data error summed in quadrature) to clearly identify a geophysical signal. Relative to surface water Δ 14 C, the depletion of preindustrial thermocline Δ 14 C is estimated to be ~10‰, as thermocline Δ 14 C is estimated to be −51‰ [32] and the south-shore coral Δ 14 C is on average −40‰. For biennial sampling, this translates into an upper bound on observable changes in water mass renewal of ~0.2 per year or 20%. To detect such a change, the background replacement rate of 16% per year would have to double. Sustained exchange perturbations over multi-annual to decadal time scales are constrained within a correspondingly smaller range of water mass renewal rates. The strong coherence and similar amplitude of atmosphere and surface water Δ 14 C variations on decadal time scales leaves little room for substantial low-frequency variability in surface water–thermocline exchange, assuming that exchange with other low Δ 14 C reservoirs, such as the GS and slope water, do not co-vary and cancel out surface water Δ 14 C variations. Despite previous findings [11] , variations in atmospheric Δ 14 C appear to be the controlling factor for Δ 14 C of surface waters in the central and southern Sargasso Sea. The south-shore coral, representative of conditions in the Hydrostation S region, demonstrates that ventilation rates in the central and southern Sargasso Sea have not been highly variable over the past 200 years. Therefore, although ventilation is certainly supplying low Δ 14 C water to the surface, the amount supplied per year has not changed within a factor of 2 (upper bound) during that time. Although the magnitude of EDW formation in the northern Sargasso Sea is known to co-vary with intensity and phase of the NAO [10] , we show that ventilation in the central and southern Sargasso Sea has not varied, neither during periods of large changes in NAO intensity nor during the colder conditions at the end of the LIA. Therefore, if a significant portion of anthropogenic carbon is being absorbed into the ocean interior in this region, it does not appear to be returning to the surface at a variable rate with time. Overall, the physical and biogeochemical processes currently established in the southern and central Sargasso Sea [5] , including rates of heat exchange, carbon sequestration and primary production due to nutrients supplied by ventilation, appear to be more stable over longer time scales than previously estimated, even in the face of changing climatic conditions. Coral sub-sampling and analysis Corals of Diploria labyrinthiformis were collected from surface waters (at a depth of 16 m) south of Johns Smith Bay, Bermuda ( Fig. 1 ). Biennial (2-year) samples were identified from X-radiographs and cut using a diamond wire saw. The Δ 14 C measurements were conducted using accelerator mass spectrometry at the University of California, Irvine. The accelerator mass spectrometry measurements have an uncertainty of ±2.5‰. The δ 13 C measurements were made on parallel samples using a Finnigan MAT 253 coupled to a Kiel carbonate device at Woods Hole Oceanographic Institution, with an uncertainty of ±0.03‰. The Δ 14 C values were then used to compare water mass renewal rates in the Sargasso Sea, using an inverse model [11] , [25] . How to cite this article: Goodkin, N. F. et al . Two centuries of limited variability in subtropical North Atlantic thermocline ventilation. Nat. Commun. 3:803 doi: 10.1038/ncomms1811 (2012).